Hybrid sensors based on colour centres in diamond and piezoactive layers The ability to measure weak signals such as pressure, force, electric field and temperature with nanoscale devices and high spatial resolution offers a wide range of applications in fundamental and applied sciences. Here we present a proposal for a hybrid device composed of thin film layers of diamond with colour centres and piezoactive elements for the transduction and measurement of physical signals. The magnetic response of a piezomagnetic layer to an external stress or a stress induced by a signal is shown to affect significantly the spin properties of nitrogen-vacancy centres in diamond. Under ambient conditions, realistic environmental noise and material imperfections, we show that this hybrid device can achieve significant improvements in sensitivity over the pure diamond-based approach in combination with nanometre-scale spatial resolution. Furthermore, the proposed hybrid architecture offers novel possibilities for engineering strong coherent couplings between nanomechanical oscillator and solid state spin qubits. The sensitive measurement of signals, such as force, pressure, electric field, temperature, with high spatial resolution possesses a wide range of applications in physics, nano science, engineering and the life sciences. Conventional methods—for example, for pressure detection—can usually operate at length scales down to the micron scale. Going beyond this regime while retaining highest sensitivity represents a significant challenge. Recently, the negatively charged nitrogen-vacancy (NV) centre in diamond [1] has been established as a highly sensitive room-temperature nanoscale probe for magnetic [2] , [3] and electric fields [4] as well as temperature [5] , [6] , [7] building on the strength of the excellent coherence properties of the NV-centre electron spin. The operational principle of such kind of pure diamond quantum sensor is based on the fact that a magnetic/electric field or temperature change will directly affect the spin properties of the NV centre, which can then be detected by optical means. The effect of pressure acting on a diamond lattice, for example, leads to the coupling between the orbital and spin dynamics of the NV centre. This offers a method to measure very high pressure with a sensitivity better than existing techniques [8] . At room temperature, however, the coupling between the strain of the diamond lattice and the ground state manifold of the NV-centre spin is insufficient for measuring a sub-MPa pressure. In this work, we propose a hybrid device that combines an NV-centre quantum sensor in diamond with a surface layer of piezomagnetic material as a signal transducer. The growth of ultrapure isotopically modified diamond and subsequent nitrogen implantation make it possible to engineer NV centres close to the diamond surface [9] , [10] , [11] (see also Müller, C. et al ., manuscript in preparation) and therefore in close proximity to the piezomagnetic material layer. This allows for the detection of changes in the stray magnetic field [3] , [12] , [13] , [14] , [15] , [16] generated by the piezomagnetic material because of an external stress. We find that the effect of pressure on the NV-centre spin can be amplified by three orders of magnitude when compared with its direct effect on the diamond [8] . However, as the NV centre lies close to the magnetic material, the magnetic noise is also expected to become more significant and deteriorate the measurement sensitivity. We analyse the sensitivity of such a hybrid diamond–piezomagnetic device for the measurement of stress (force) with detailed numerical studies, and show that a sensitivity of (tens of ) can be achieved for the measurement of pressure (force) under ambient conditions with state-of-the-art experimental capabilities by choosing appropriate control parameters. In combination with piezoelectric and thermally sensitive elements, our proposed hybrid piezomagentic-NV approach also provides a new method for the measurement of electric field and temperature with an improved sensitivity as compared with standard diamond NV sensors [4] , [5] , [6] , [7] . The model We consider a system (see Fig. 1a ) made up of a diamond layer grown on the surface of a thin piezomagnetic film such as Tb 0.27 Dy 0.73 Fe 2 (Terfenol-D) that exhibits a high magnetostrictive effect. The surface area of the piezomagnetic film can be reduced to a designed size by subsequent selective etching. The NV centre is implanted in the diamond layer with a depth denoted as d from the interface between the magnetic film and diamond. The ground 3 A 2 level of the NV-centre spin exhibits a zero field splitting of D =2.87 GHz between the m s =0 and m s =±1 spin sublevels. 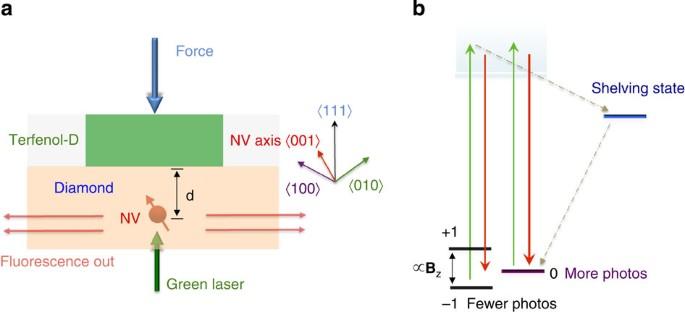Figure 1: A hybrid quantum sensor of a diamond layer with colour centres implanted and a piezoactive layer. (a) The model hybrid system of diamond (brown) and piezomagnetic film (green). The application of a uniaxial stress induces the change of the magnetostrictive behaviour of the piezomagnetic film, which produces a stray magnetic field change measured by the NV centre implanted in diamond. (b) The energy level structure of a single NV centre. The ground spin sublevels (±1, 0) can be initialized and readout via side-collection spin-dependent photoluminescence17, and the coherent control of the NV spin is implemented with a microwave field. The spin Hamiltonian, including the strain effect of the diamond lattice and the Zeeman interaction with a magnetic field, is given by Figure 1: A hybrid quantum sensor of a diamond layer with colour centres implanted and a piezoactive layer. ( a ) The model hybrid system of diamond (brown) and piezomagnetic film (green). The application of a uniaxial stress induces the change of the magnetostrictive behaviour of the piezomagnetic film, which produces a stray magnetic field change measured by the NV centre implanted in diamond. ( b ) The energy level structure of a single NV centre. The ground spin sublevels (±1, 0) can be initialized and readout via side-collection spin-dependent photoluminescence [17] , and the coherent control of the NV spin is implemented with a microwave field. Full size image where γ =28 MHz mT −1 is the electron gyromagnetic ratio, is the combination of the stray magnetic field B p generated by the piezomagnetic film and the applied external magnetic field along the NV axis (that connects the nitrogen and vacancy sites). The effect of strain on the NV centre, as quantified by E , induces ground-state spin sublevel mixing and is usually much smaller (on the order of MHz) than the energy splitting of the ground-state triplet. The zero-field splitting D is slightly affected by the stress because of pressure σ , with a gradient of about d D ( σ )/d σ ~\n15 kHz/MPa at room temperature [8] . In this work, we will be mostly interested in the case of a weak (sub MPa) pressure, and therefore such a direct effect of stress in the diamond lattice on the NV spin is negligible. The coupling strength between an electric field and the NV ground-state spin is also negligible in the present model [18] . The spin-dependent fluorescence of an NV centre (see Fig. 1b ) provides an efficient mechanism to optically initialize and readout the ground-state spin, and to perform optically detected magnetic resonance (ODMR) measurements in the ground state. The resonance frequencies ω ±1 in the ODMR spectra corresponding to the electronic transitions from the spin sublevel m s =0 to ±1, respectively, depend on the magnetic field acting on the NV centre. The piezomagnetic material consists of magnetic domains, in which the magnetization is uniform M k = M S m k , where M S is the saturation magnetization of the material, and with being the direction cosines with respect to the crystal axes. The response of the piezomagnetic materials that have large magnetostriction, such as Terfenol-D, leads to a change of the magnetization directions of magnetic domains, and in turn of the stray magnetic field [19] , [20] that affects the spin properties of an NV centre. ODMR response to a uniaxial stress To estimate the stress-induced change of the stray magnetic field and the corresponding magnetic noise acting on the NV-centre spin, we perform micromagnetic simulation using Landau–Lifshitz–Gilbert equation. We first calculate the steady state of Terfenol-D film (characterized by the parameters in Supplementary Table 1 ) under varying stress by using the Landau–Lifshitz–Gilbert micromagnetic dynamic equation ( Supplementary Equation 1 in Supplementary Note 1 ). To account for the thermal fluctuation at room temperature, we add a random thermal fluctuation field H th to the effective magnetic field H k in the micromagnetic dynamic equation, and describe the thermal field H th as a Gaussian random process with the strength determined by the fluctuation-dissipation theorem [21] , [22] , [23] , see Supplementary Note 1 . We apply an external magnetic field along the NV axis, which is assumed to be in the ‹001› direction and set it as the z axis, and consider a stress along the ‹111› direction with respect to the crystal axes in the piezomagnetic material (see Supplementary Note 2 ), along which it has the largest magnetostriction coefficient, see Supplementary Table 1 . By solving the Langevin equation using the stochastic Heun scheme [24] , we calculate the effective magnetic field acting on the NV centre and observe a prominent resonance frequency shift in the ODMR spectra, see Fig. 2 . The shift of Δ= ω +1 − ω −1 is approximately linear with the stress, and the gradient is about dΔ/d σ ~\n17 MHz/MPa for the NV centre at a depth of d =15 nm, which is about three orders of magnitude larger than the shift of the zero-field splitting parameter D under a direct pressure [8] . We remark that the stress-induced frequency shift of the NV centre can be further improved by optimizing the dimension of the piezomagnetic film and the depth of the NV centre. For example, we find that dΔ/d σ ~\n36 MHz/MPa for d =10 nm, although the magnetic noise may also increase (see Supplementary Note 3 ). Besides the frequency gradient dΔ/d σ , the shot-noise-limited sensitivity also depends on the coherence time of the NV centre, which we will determine in the following section. 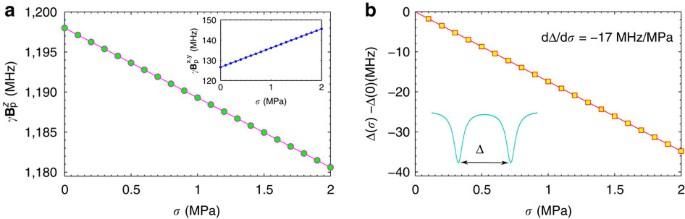Figure 2: The response of the NV centre spin to a uniaxial stress. (a) The stray field component parallel () and perpendicular (, inset) to the NV axis. (b) The separation Δ between two resonance frequencies in the ODMR spectra as a function of the stressσ. The value of Δ is 15.55 GHz forσ=0. The dimension of the Terfenol-D film is chosen as (15 nm)3, and the distance from the NV centre to the interface isd=15 nm. The applied external magnetic field isB0=2,350 G along the ‹001› direction, and the stress is along the ‹111› direction. The temperature is 300 K. Figure 2: The response of the NV centre spin to a uniaxial stress. ( a ) The stray field component parallel ( ) and perpendicular ( , inset) to the NV axis. ( b ) The separation Δ between two resonance frequencies in the ODMR spectra as a function of the stress σ . The value of Δ is 15.55 GHz for σ =0. The dimension of the Terfenol-D film is chosen as (15 nm) 3 , and the distance from the NV centre to the interface is d =15 nm. The applied external magnetic field is B 0 =2,350 G along the ‹001› direction, and the stress is along the ‹111› direction. The temperature is 300 K. Full size image Noise power spectrum and measurement sensitivity At a finite temperature, the thermal fluctuation of the piezomagnetic film induces a fluctuating magnetic field acting on the NV-centre spin, which gives rise to the ODMR linewidth broadening and thereby the decay of spin coherence. Using a pulsed sensing scheme, the NV spin is first prepared into a coherent superposition state by applying a microwave driving field H d = Ω [cos( ω +1 t )|+1›‹0|+cos( ω −1 t )|−1›‹0|] +h.c. for a pulse duration t π/2 = π / Ω . We remark that by choosing the spin sublevels m s =−1 and +1 to encode quantum coherence, the temperature instability [5] , [6] , [7] and electric noise will shift the energies of these two levels equally (Supplementary Equation 10 in Supplementary Note 4 ), and thus would not cause dephasing. The ideal evolution of the NV spin is . The electronic spin coherence time of an NV centre in isotopically engineered diamond can exceed 100 μs even at room temperature [25] , [26] ; thus, the dominant magnetic noise in the present model arises from the fluctuation in the magnetic material (see Supplementary Note 4 for the analysis of other noises). By solving the stochastic Langevin equation including the thermal random field to the simulation of micromagnetic dynamics, we obtain the time correlation function R ζ ( t )=‹ B ζ ( t ) B ζ (0)›−‹ B ζ ( t )›‹ B ζ (0)› of the magnetic noise from the Terfenol-D film, where ζ = x , y , z represents the field component along the x , y , z directions. In Fig. 3a,b , we plot the noise correlation functions, which show a fast decay on a timescale on the order of nanoseconds. The noise correlation functions can be fitted by R ζ ( t )= R ζ (0) e − tξ cos ( ω 0 t ), where ξ −1 characterizes the the correlation time of the magnetic noise, and it depends on the Gilbert damping constant α d of the piezomagnetic material (for Terfenol-D, the value of α d ~\n0.1 (ref. 27 ), see Supplementary Note 5 for detailed discussion). The oscillatory feature of the noise correlation function is related to the precession of magnetic domains, whose frequency ω 0 is dependent on the applied external magnetic field B 0 and the demagnetization field among magnetic domains. The latter is determined by the parameters of the piezomagnetic material. 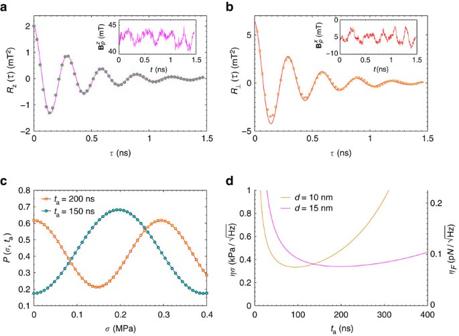Figure 3: Properties of the magnetic noise and the measurement sensitivity of the hybrid sensor at room temperature. (a,b) The time correlation function of the magnetic noise (the parallel componentRz(τ) (a) and the perpendicular conponentR⊥(τ)=[Rx(τ)+Ry(τ)]/2 (b) with respect to the NV axis) emanating from the magnetic material. The symbols, circle inaand squares inb, are the results from numerical simulations, and the curves are fitting functionsRζ(t)=Rζ(0)e−tξcos(ω0t) with the characteristic parametersω0=(2π) 3.38 GHz andξ=2.8 GHz (see equation (2)). The inset shows one random trajectory of the fluctuating magnetic field acting on the NV-centre spin due to the thermal fluctuation in the magnetic material. (c) Example of simulated signal as a function of the applied uniaxial stressσat the interrogation timeta. The signal contrast decreases for the largertadue to the decoherence caused by the magnetic noise. (d) The shot-noise-limited sensitivity for the measurement of stress (and force) within the total experiment time of 1 s as a function of interrogation timeta(see equation (4)). The value of is 0.3, the NV spin preparation and readout time istp=600 ns. The other parameters are the same as inFig. 2. The noise power spectrum is obtained from the Fourier transformation of the correlation function as Figure 3: Properties of the magnetic noise and the measurement sensitivity of the hybrid sensor at room temperature. ( a , b ) The time correlation function of the magnetic noise (the parallel component R z ( τ ) ( a ) and the perpendicular conponent R ⊥ ( τ )=[ R x ( τ )+ R y ( τ )]/2 ( b ) with respect to the NV axis) emanating from the magnetic material. The symbols, circle in a and squares in b , are the results from numerical simulations, and the curves are fitting functions R ζ ( t )= R ζ (0) e − tξ cos( ω 0 t ) with the characteristic parameters ω 0 =(2π) 3.38 GHz and ξ =2.8 GHz (see equation (2)). The inset shows one random trajectory of the fluctuating magnetic field acting on the NV-centre spin due to the thermal fluctuation in the magnetic material. ( c ) Example of simulated signal as a function of the applied uniaxial stress σ at the interrogation time t a . The signal contrast decreases for the larger t a due to the decoherence caused by the magnetic noise. ( d ) The shot-noise-limited sensitivity for the measurement of stress (and force) within the total experiment time of 1 s as a function of interrogation time t a (see equation (4)). The value of is 0.3, the NV spin preparation and readout time is t p =600 ns. The other parameters are the same as in Fig. 2 . Full size image As the correlation time of the magnetic noise is much shorter than the coherence time of the NV spin, we can describe the NV spin dynamics under the environmental noise by a quantum master equation as derived in Supplementary Note 6 . The fluorescence measurement of the state m s =0 population after an interrogation (that is, free evolution) time t a and a subsequent ( π /2) pulse is where the dephasing and relaxation coefficients χ || ( t )=exp (−4 t S z (0)), χ ⊥ ( t )=exp(− t S ⊥ ( ω −1 )/2) are determined by the magnetic noise power spectrum, where S ⊥ =( S x + S y )/2. To obtain the optimal measurement sensitivity, we choose t a such that the signal has the maximum absolute slope with respect to the stress, namely |sin( t a Δ)|=1. The shot-noise-limit sensitivity for the measurement of stress within a total experiment time T is obtained as follows where t p is the preparation and readout time in each experiment run, accounts for the NV state initialization, readout efficiency and the signal contrast. The value of can exceed 0.3 by improving the collection efficiency using a plasmonic or optical waveguide [17] , [28] . The quantity η σ , , T characterizes the smallest change in the stress that can be identified within the total experiment time T . By choosing a larger interrogation time of t a , it is possible to improve the slope of the signal (see equation (4)) while in the mean time the NV-centre spin would suffer more from the magnetic noise. This implies an optimal interrogation time to achieve the best sensitivity. In Fig. 3c,d , we plot the simulated fluorescence signal at two different interrogation times, and the shot-noise-limit sensitivity for the measurement of stress (force), which can achieve and , respectively. Such a sensitivity is close to the one achieved by atomic force spectroscopy (see, for example, ref. 29 ), while requiring less stringent operating environment and being more robust. We remark that the sensitivity may be further improved by optimizing the dimension of the hybrid system and using an array of NV centres. Electric field and temperature measurement Although the NV centre has been used to measure electric field [4] and temperature [5] , [6] , [7] , the sensitivity is largely limited by the efficiency of the direct coupling between the NV-centre spin and electric field (temperature). Here we propose to combine the hybrid diamond and piezomagnetic device with a piezoelectric element island on a substrate to measure electric field (see Supplementary Note 7 ). An electric field E induces a strain ε = ε e · E of the piezoelectric element island, which generates a stress σ = ε · Y acting on the attached piezomagnetic layer where Y denotes the Young’s modulus of the piezoelectric material. For a piezoelectric island that has large piezoelectric constants, such as Pb[Zr x Ti 1− x ]O 3 and simultaneously low optical absorption [30] , the electric-field-induced strain can be as large as ε e ~\n0.0002 (MV/m) −1 , the corresponding Young’s modulus is Y ~\n10 5 MPa (ref. 31 ). The mediated coupling coefficient between the NV spin (at a depth of 15 nm) and the electric field is thus dΔ/d E =( ε e · Y )(dΔ/d σ )=34 kHz (V/cm) −1 , as compared with the direct coupling coefficient of ~\n10 Hz (V/cm) −1 (ref. 18 ). The sensitivity for the measurement of electric field thus reaches η e = η σ /( ε e · Y ). As the coupling between the NV centre and the electric field is rather weak compared with the magnetic noise, and because the charge noise decreases rapidly with the distance from the NV centre to the piezoactive layer [32] , at a distance of, for example, 10–15 nm, it is at least three orders of magnitude smaller than the magnetic noise effect considered above (see Supplementary Note 4 ). In the mean time, the charge noise in an isotopically engineered diamond [25] is also negligible. The sensitivity for the pressure measurement therefore implies the sensitivity for the measurement of electric field as high as , which significantly exceeds the sensitivity of by a pure diamond NV sensor [4] . This sensitivity would allow for the detection of the electric field produced by a single elementary charge at a distance from the NV-spin sensor of ~\n8 μm in around 1 s , going beyond the single electron spin detection capacity of magnetic resonance force microscopy [33] , and thus opens the possibility of remote sensing of a single charge under ambient conditions. We remark that a similar sensitivity can be achieved in an NV-diamond electrically induced transparency device, which however requires an ensemble of NVs and liquid–nitrogen temperature [34] . In a similar way, it is possible to combine the hybrid diamond and piezomagnetic device with a thermally sensitive element island on a substrate to measure temperature (see Supplementary Note 7 ). A change of temperature induces the expansion of the thermally sensitive element island as characterized by its thermal expansion constant ε T , which can be as high as 2.3 × 10 −5 K −1 (aluminium). The thermal expansion produces a stress acting on the attached piezomagnetic layer as σ T =( ε T · T ) Y , where Y denotes the Young’s modulus of the thermally sensitive material, for example, Y =7 × 10 4 MPa (aluminium). Thus, the response of the resonance frequency of an NV centre at a depth of 15 nm is dΔ/d T =( ε T · Y )(dΔ/d σ )=27 MHz K −1 , which represents significant improvement over the value dΔ/d T ~\n74 kHz K −1 of a pure diamond NV sensor [35] . The sensitivity for the measurement of temperature can reach and does not require an interrogation time of millisecond [5] , [6] , [7] . The proposed that diamond–piezomagnetic hybrid sensor combines high sensitivity under ambient conditions with nanometre-scale dimensions improving the sensitivity of standard diamond sensing devices by up to three orders of magnitude. The high spatial resolution is achieved, thanks to the atomic size of the NV centre and the ability for positioning it with high accuracy [5] , [9] , [10] , [11] , [36] , [37] , [38] in nanoscale diamond. Special attentions to, for example, surface preparation and heating control would be necessary for an even better sensitivity. Such a device can find a wide range of applications for measuring force and pressure, electric field and temperature changes under ambient conditions, such as protein folding and DNA stretching (see Supplementary Note 8 ) in life science [39] . Furthermore, it offers a precise way to determine the short-range forces between two plates (or spheres) and may have implications for the study of fundamental quantum physics phenomena such as an accurate description of the Casimir effect [40] or non-Newtonian forces (for example, Yukawa-type forces) where forces have to be measured at smallest distances (below 100 nm) [41] . It also provides a possible way to detect an elementary charge (electron) over a distance of micrometres. Besides its application in signal transduction and precision measurement, it may also find applications in spin and mechanical oscillator hybrid systems. A hybrid diamond–piezomagnetic (film) mechanical nanoresonator can significantly enhance the coherent coupling between its vibrational mode and NV electronic spins in diamond [42] , [43] , and thereby boost the phonon-mediated effective spin–spin interactions. This would allow fast mechanical control of spin qubits and efficient phonon cooling by an NV centre [42] , [43] , [44] , [45] , [46] , [47] and would facilitate the generation of spin squeezing at room temperature, which can be used as a resource for magnetometry and phonon-mediated quantum information processing. The extension of the present model to arrays may find applications in tactile imaging [48] and instantaneous pressure visualization by interactive electronic skin [49] . The proposed device may also find applications in nanoscale surface characterization, for example, in read/write heads of hard disks where the enhanced sensitivity to magnetic fields in combination with nanoscale spatial resolution may significantly increase the characterization speed (by decreasing the number of repetitive interrogation times while sustaining a readout precision criteria) which is a crucial constraint in industrial applications. How to cite this article: Cai, J. et al . Hybrid sensors based on colour centres in diamond and piezoactive layers. Nat. Commun. 5:4065 doi: 10.1038/ncomms5065 (2014).